Fundamental origins and limits for scaling a maternal morphogen gradient Tissue expansion and patterning are integral to development; however, it is unknown quantitatively how a mother accumulates molecular resources to invest in the future of instructing robust embryonic patterning. Here we develop a model, Tissue Expansion-Modulated Maternal Morphogen Scaling (TEM 3 S), to study scaled anterior–posterior patterning in Drosophila embryos. Using both ovaries and embryos, we measure a core quantity of the model, the scaling power of the Bicoid (Bcd) morphogen gradient’s amplitude n A . We also evaluate directly model-derived predictions about Bcd gradient and patterning properties. Our results show that scaling of the Bcd gradient in the embryo originates from, and is constrained fundamentally by, a dynamic relationship between maternal tissue expansion and bcd gene copy number expansion in the ovary. This delicate connection between the two transitioning stages of a life cycle, stemming from a finite value of n A ~3, underscores a key feature of developmental systems depicted by TEM 3 S. Scaling of biological activities with organismal size is a general property of life [1] ; however, it is actively debated whether all life forms and biological activities follow a single universal scaling relationship [2] , [3] , [4] , [5] , [6] , [7] . From the perspective of developmental biology, scaling is about proportionality of tissue/organ size to the overall body size, which is one of the most intriguing but poorly understood features of animal development [8] , [9] , [10] . Two aspects of the developmental scaling problem, formation of scaled patterns and expansion of specified tissues, have been investigated intensively [11] , [12] , [13] , [14] , [15] , [16] , [17] , [18] , [19] , [20] . To provide a unified perspective suitable for evaluating diverse systems at different levels, we can define the relationship between tissue specification (patterning) and tissue expansion (growth) of a given developmental system based on how they are connected temporally within a time period of interest. These two events can take place either concurrently or with one preceding the other, representing three basic types of temporal relationships or temporal logics ( Fig. 1a ). In logic a , such as the Drosophila wing disc, tissue patterning and expansion are concurrent events that could also (but do not have to) be coupled mechanistically [21] , [22] . In logic b , such as the increase in an animal’s muscle mass, patterning of a tissue precedes its expansion [13] , [20] . In logic c , such as the Drosophila embryo, patterning takes place when size has been pre-determined [23] . 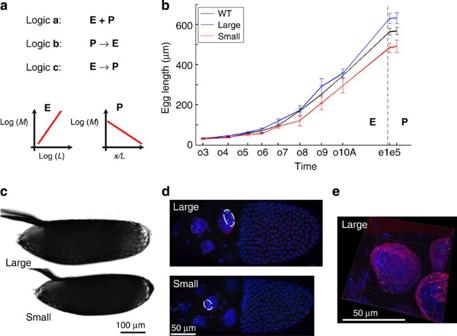Figure 1: Investigating tissue expansion properties during oogenesis inDrosophila. (a) Diagrams depicting three basic temporal logics governing the relationships between tissue expansion (E) and patterning (P) within a time period of interest. A symbolic plot capturing each system’s fundamental feature is shown. For the depicted systemE, whereMrefers to a given type of molecules (for example, mRNA or protein) that accumulate in quantity in relation to the 1D size,L, of the system, the slope shown is the scaling power,n, of the molecules. For the depicted systemP, whereMrefers to morphogen molecules that form an exponential concentration gradient along the normalized length,x/L, of the patterning system, the slope shown is −Γ, negative of the system attribute (see Results for additional details). (b) Measured lengths of egg chambers and embryos. WT, Large and Small denotew1118, large- and small-egg inbred lines, respectively (shown in black, blue and red, respectively). Error bars are s.d.’s and sample numbers are 50 (embryos) or four or more (egg chambers) for each of the three lines at each of the stages shown. Student’st-tests suggest significant between-strain differences in lengths (Pvalues<0.05) as early as oogenesis stage 6. (c,d) Freshly laid eggs (c) or stage-10A egg chambers (d) from inbred lines. White circle indmarks the cluster of the detectedbcdDNA FISH dots (green) within a nurse cell nucleus (DAPI in blue; WGA in red; see Methods). (e) Higher magnification of a stage-10A egg chamber. Scale bars, 100 μm (forc) and 50 μm (ford,e). Figure 1: Investigating tissue expansion properties during oogenesis in Drosophila . ( a ) Diagrams depicting three basic temporal logics governing the relationships between tissue expansion ( E ) and patterning ( P ) within a time period of interest. A symbolic plot capturing each system’s fundamental feature is shown. For the depicted system E , where M refers to a given type of molecules (for example, mRNA or protein) that accumulate in quantity in relation to the 1D size, L , of the system, the slope shown is the scaling power, n , of the molecules. For the depicted system P , where M refers to morphogen molecules that form an exponential concentration gradient along the normalized length, x / L , of the patterning system, the slope shown is − Γ , negative of the system attribute (see Results for additional details). ( b ) Measured lengths of egg chambers and embryos. WT, Large and Small denote w 1118 , large- and small-egg inbred lines, respectively (shown in black, blue and red, respectively). Error bars are s.d.’s and sample numbers are 50 (embryos) or four or more (egg chambers) for each of the three lines at each of the stages shown. Student’s t -tests suggest significant between-strain differences in lengths ( P values<0.05) as early as oogenesis stage 6. ( c , d ) Freshly laid eggs ( c ) or stage-10A egg chambers ( d ) from inbred lines. White circle in d marks the cluster of the detected bcd DNA FISH dots (green) within a nurse cell nucleus (DAPI in blue; WGA in red; see Methods). ( e ) Higher magnification of a stage-10A egg chamber. Scale bars, 100 μm (for c ) and 50 μm (for d , e ). Full size image Our current work concerns temporal logic c . In Drosophila , patterning along the anterior–posterior (AP) axis of the embryo is instructed by the maternal morphogen gradient Bicoid (Bcd) [24] , [25] , [26] , [27] , [28] . A well-recognized feature of this system is the robust and scaled patterning outcome [11] , [12] ; however, its underlying mechanisms remain a topic of active investigation. Our recent studies have led to the documentation that the Bcd morphogen gradient in Drosophila melanogaster embryos possesses scaling properties [14] , [23] , [29] . We found that a general property of the embryo relevant to Bcd gradient scaling is that the amount of maternally deposited bcd mRNA is correlated with embryo size [23] , [29] . However, the precise origin of such a correlation remains unknown. In addition, although one of our documented within-species scaling mechanisms has a resemblance to a between-species scaling mechanism [29] , [30] , it represents a special case involving abnormal bcd mRNA localization in the embryo. Thus, we are currently lacking a unified mechanistic view of the maternal origins and evolutionary conservation of Bcd gradient scaling in the embryo. In this report we establish, and experimentally advance, a framework designed to evaluate the origins and limits of Bcd gradient scaling within a species. Our framework is referred to as the Tissue Expansion-Modulated Maternal Morphogen Scaling (TEM 3 S) model. This model unifies specifically and quantitatively the properties and events of maternal tissue expansion and scaled embryonic patterning under temporal logic c . We perform independent measurements to estimate a core quantity of this model, the scaling power of Bcd gradient’s amplitude n A . We also perform measurements to directly evaluate model-derived predictions in the embryo. We show that, in addition to connecting the events that take place in two distinct stages of Drosophila life cycle, the TEM 3 S model also provides a unified view of the two distinct scenarios of Bcd gradient scaling (that is, within-species versus across-species) from an evolutionary perspective at a mechanistic level. The TEM 3 S model We establish a general framework of biological scaling in a developmental system that follows temporal logic c ( Fig. 1a ). Here tissue expansion takes place in a biological entity referred to as system E , while patterning takes place in a distinct (but connected by the life cycle) entity referred to as system P . We base our model on the Drosophila morphogen gradient of Bcd. Thus, tissue expansion in our model refers specifically to the growth of an egg chamber in the ovary of the mother (system E ) and scaled spatial patterning is a property that is specific to the future embryo (system P ). One of our objectives is to build a unified conceptual framework within which we can compare model-derived predictions with observed properties of the actual biological systems. In our theoretical discussions that are further detailed in Supplementary Notes 1–4 , we may on occasions choose to use parameter values that are idealistic, but they are consistent with the actual biological system in hand. Importantly, our general conclusions about the expected behaviour of developmental systems depicted by the TEM 3 S model do not depend on particular parameter values chosen for analysis. In previous studies of the Bcd morphogen gradient, a patterning system’s length L is usually treated as a given value when the gradient behaviours are evaluated [31] , [32] , [33] , [34] , [35] , [36] , [37] , [38] . In our discussion, we treat L as a property that is inherited specifically from system E . Under temporal logic c , L is predetermined by system E , representing a variable that is independent of space or time in system P . This feature makes the Bcd gradient different from morphogen systems that follow other temporal logics. Since our discussion focuses on scaling, we express a given position x along the length of system P as a relative value ξ = x / L . The TEM 3 S model formalizes the scaling feature of patterning by stating that a morphogen gradient possesses properties necessary for it to achieve a performance objective in system P . Performance objective is defined as attaining one (or more) relative position ξ , at which morphogen concentration M is insensitive to fluctuations in L . This necessitates a search for a solution(s) of ξ to the first-order partial differentiation with respect to L being zero as We denote the solution ξ = ξ C as the critical position of system P . This solution could be a function of t (that is, scaling is time-dependent); however, by definition it is independent of L . To be a realistic value, ξ C must be within the physical boundary [0 1] of system P . The Bcd gradient profile may be approximated by an exponential function [11] , [26] . Here we consider a two-parameter model of an exponential morphogen gradient that is stable over time, . In an idealized 1D model based on synthesis, diffusion and decay, this gradient represents the steady-state morphogen concentration, where A = J /( Dω ) 1/2 and Γ = L /( D / ω ) 1/2 , and J is the morphogen production rate from a point source at ξ =0, D is the diffusion constant and ω is the first-order rate constant of decay (see Supplementary Figs 1–4 and Supplementary Notes 1–4 for additional considerations). In this two-parameter model, either the amplitude A or the slope measurement Γ (or both) could be a quantity related to L . For our study, we define scaling power, , as the normalized derivative of a biological quantity Q with respect to that of the system length L . If n Q can be approximated to a finite constant value with respect to L , we have a power-law relationship . If Γ is independent of L , that is, n Γ =0, it is possible for all positions to satisfy equation (1). If n Γ ≠0, there is only one solution to equation (1), ξ C = n A / Γ n Γ . By definition, this solution determines the critical position, at which M is insensitive to fluctuations in L . Under the condition that diffusivity and decay of morphogen molecules are properties intrinsic to a given species and thus insensitive to L , that is, n Γ =1, we have Equation (2) shows that, for a stable exponential gradient whose slope is independent of L , the performance objective of attaining ξ C could be achieved only if Γ is properly matched by the scaling power of a morphogen gradient’s amplitude n A ( Supplementary Fig. 1 and Supplementary Note 1 ). For purposes of perspective and convenience, we refer to Γ , which quantifies the length of system P in a relative term, as the system attribute. In biochemical terms, Γ could be viewed as a constant that exists for a given species and this constant can be evaluated through experimental measurements in the embryos. Equation (2) provides a general expression of the TEM 3 S model. It states straightforwardly that the behaviour of system P with regard to the existence and location of its critical position (defined as ξ C ) is determined by the fundamental properties that connect system E to system P (as encapsulated by n A —see below) and the length of system P in relation to the gradient’s length scale (as signified by Γ ). A dynamic framework connecting system E to system P In the TEM 3 S model, both the 1D size L and the scaling power of the morphogen gradient’s amplitude n A in system P can be viewed as inherited properties in the sense that they are derived from system E that has ceased to exist but has been physically transitioned into system P . To formally link systems E and P , we develop a quantitative framework that describes the dynamic relationship between size and scaling power ( Supplementary Note 2 ). In this framework, the morphogen protein in the embryo (system P ) is the end product in a chain of linear-forward transitions between molecular species that originate from the egg chamber in the ovary (system E ): gene→mRNA→protein. Here morphogen gene copies and morphogen protein molecules are unique to systems E and P , respectively, and morphogen mRNA is the only species that can exist in both systems. As an egg chamber expands its size during oogenesis, morphogen gene copies undergo endoreplication (in nurse cells) and are used as templates for mRNA production (see experimental data below). Using first-order rate constants to describe dynamic tissue growth and chemical reactions, we can deduce that (see Supplementary Note 2 ), where n 1 , n 2 and n 3 are the scaling powers of each of the molecular species (gene, mRNA and protein, respectively) in the chain with respect to the length of a corresponding biological entity, and j 1 and k 1 are first-order rate constants for the expansions of, respectively, morphogen gene copy number and 1D size of a maternal entity (for example, nurse cell nucleus) during oogenesis. Equation (3) postulates a dynamic origin of the scaling power of the morphogen gradient’s amplitude n A in system P . In other words, n A , a quantity that is for system P and core to the TEM 3 S model, is defined fundamentally by the dynamic properties of system E . Thus, an experimental measurement of the quantity n A is important not only to advancing mechanisms of developmental scaling but also to understanding quantitative biological principles that govern the ‘accumulation’ and ‘consumption’ of molecular resources in connecting two stages of a life cycle. Equation (3) also states that the scaling power n A can be estimated through the use of independent methods that quantify each of the three molecular species in the linear chain, a postulate to be evaluated directly by experiments. The experimental system The Drosophila egg is derived from the maternal tissue ovary (see Methods for definition of oogenesis stages). To advance our TEM 3 S model experimentally, we first quantified growth properties of the egg chamber in the ovary. In addition to w 1118 as the wild-type (WT), we used two inbred lines that had been selected to lay large or small eggs [23] , [39] . Our measurements in the ovary document that egg size divergence between these two lines originates from oogenesis ( Fig. 1b–d ). Towards quantifying scaling powers during oogenesis, we established whole-mount procedures for the ovary (see Methods and Supplementary Table 1 ). We used DNA fluorescent in situ hybridization (FISH) to quantify individual gene loci (such as bcd ), DAPI staining to quantify bulk nuclear DNA and wheat germ agglutinin (WGA) staining to visualize the nuclear envelope ( Fig. 1d,e ). Our whole-mount tissues were processed to maximally preserve their native spatial features. In addition, our confocal imaging was performed within a documented linear range ( Supplementary Fig. 5 ). A growing egg chamber consists of one oocyte, 15 nurse cells and thousands of follicle cells [40] , [41] , [42] , [43] . Nurse cells and follicle cells provide external signals, nutrients and other materials to the oocyte that will become the future egg. Our primary interest of the current work is in nurse cells because it is these cells that produce bcd mRNA; however, for calibration purposes, we used follicle cells. These cells undergo three rounds of endoreplication [44] , [45] , leading to four well-resolved subpopulations with expected genome polyploidy of 2C, 4C, 8C and 16C ( Fig. 2a,b ; see Methods). Such calibrations within a given experiment ( Fig. 2c,d ) permitted us to estimate a nurse cell’s genome polyploidy or bcd gene copy number (see Fig. 2e,f for scatter plots of data from individual nurse cell nuclei). 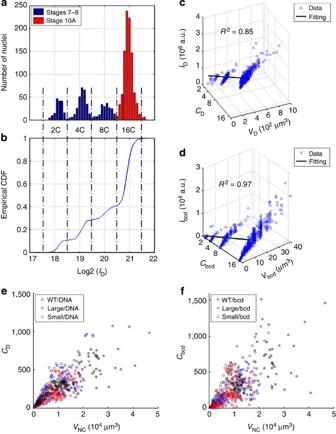Figure 2: Quantification of bulk nuclear DNA andbcdgene copy number in nurse cells. (a,b) Histogram (a) or empirical cumulative function (b) of nuclear DAPI intensity of the calibrating cells (1,649 follicle cells; see Methods). Dashed lines mark boundaries between subpopulations with the expected genome polyploidy of 2C, 4C, 8C and 16C. Datapoints from egg chambers at stages 7–9 or stage 10A are shown in blue and red, respectively. (c,d) Scatter plots showing a two-parameter linear fit,I=aC+bV, for nuclear DAPI intensity (c) orbcdDNA FISH dot intensity (d). (e,f) Scatter plots showing linear relationship between genome polyploidy equivalent (e) orbcdgene copy number (f) and nurse cell nuclear volume. Datapoints for stage 10A are marked by crosses; colour code: black, blue and red for WT, large-egg line and small-egg line, respectively. The estimated polyploidy equivalents per egg chamber at stage 10A are 5.7±0.5, 6.1±0.5 and 4.6±0.3 × 103in WT, large-egg line and small-egg line, respectively (values are mean±s.d.). They are consistent with previous estimates44considering that our calibration methods adjust for volume-dependent background intensities (see Methods). The estimatedbcdgene copy numbers are given in Main text. Consistent with the analysis of egg lengths (Fig. 1b), Student’st-tests suggest significant differences in either genome polyploidy equivalent (P-value=10−6between WT and the small-egg line, and 0.04 between WT and the large-egg line) orbcdgene copy number (Pvalue=0.04 between WT and the small-egg line, and 0.12 between WT and the large-egg line). In addition, both the average polyploidy equivalents andbcdcopy numbers of different lines show correlation with the average nurse cell nuclear volumes (Pearson correlation coefficients=1.00 and 0.99,Pvalues=0.05 and 0.09, respectively;Pvalues from Pearson coefficient calculation). Figure 2: Quantification of bulk nuclear DNA and bcd gene copy number in nurse cells. ( a , b ) Histogram ( a ) or empirical cumulative function ( b ) of nuclear DAPI intensity of the calibrating cells (1,649 follicle cells; see Methods). Dashed lines mark boundaries between subpopulations with the expected genome polyploidy of 2C, 4C, 8C and 16C. Datapoints from egg chambers at stages 7–9 or stage 10A are shown in blue and red, respectively. ( c , d ) Scatter plots showing a two-parameter linear fit, I = aC + bV , for nuclear DAPI intensity ( c ) or bcd DNA FISH dot intensity ( d ). ( e , f ) Scatter plots showing linear relationship between genome polyploidy equivalent ( e ) or bcd gene copy number ( f ) and nurse cell nuclear volume. Datapoints for stage 10A are marked by crosses; colour code: black, blue and red for WT, large-egg line and small-egg line, respectively. The estimated polyploidy equivalents per egg chamber at stage 10A are 5.7±0.5, 6.1±0.5 and 4.6±0.3 × 10 3 in WT, large-egg line and small-egg line, respectively (values are mean±s.d.). They are consistent with previous estimates [44] considering that our calibration methods adjust for volume-dependent background intensities (see Methods). The estimated bcd gene copy numbers are given in Main text. Consistent with the analysis of egg lengths ( Fig. 1b ), Student’s t -tests suggest significant differences in either genome polyploidy equivalent ( P -value=10 −6 between WT and the small-egg line, and 0.04 between WT and the large-egg line) or bcd gene copy number ( P value=0.04 between WT and the small-egg line, and 0.12 between WT and the large-egg line). In addition, both the average polyploidy equivalents and bcd copy numbers of different lines show correlation with the average nurse cell nuclear volumes (Pearson correlation coefficients=1.00 and 0.99, P values=0.05 and 0.09, respectively; P values from Pearson coefficient calculation). Full size image Metric expansion of nurse cell nuclei Nurse cells undergo three distinct phases of endoreplication [46] : (1) complete replication during the first five rounds to form a single polytene chromosome, (2) dispersion of the 64 chromosomes into 32 chromatid pairs and (3) additional rounds of endoreplication for each of these 32 polytene chromosomes. The bcd gene loci detected in our whole-mount FISH remain spatially clustered inside the nurse cell nucleus ( Fig. 1d,e ). Such clusters could reflect the working of ‘continued forces’ that drive, for example, homologous pairing or interactions with the nuclear architecture to restrict free expansion [47] . Alternatively, the clusters themselves could expand in a manner that is analogous to metric expansion, in which case the existence of such clusters would reflect the working of the ‘initial forces’ that restricted the dispersion step. Our results obtained from both WT ( Fig. 3a ) and the inbred lines ( Fig. 3b ) are consistent with the latter hypothesis and support a volumetric expansion after dispersion. 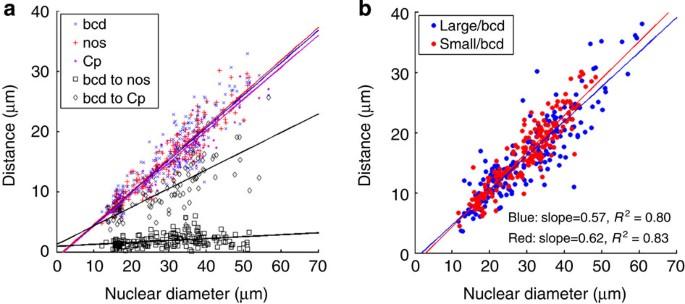Figure 3: Expansion of gene locus clusters in expanding nurse cell nuclei. (a) Scatter plots of the observed cluster size for individual gene loci (bcd,nosorCp, shown in blue, red and purple, respectively), or the observed distance between two clusters (bcd-nosorbcd-Cp, shown in black and grey, respectively), against nurse cell nuclear diameter (see Methods for definition of cluster size and distance between clusters). Data are from WT egg chambers at stages 6~10 A. Solid lines are linear fits. Blue:y=0.54x−0.92 μm,R2=0.86; red:y=0.54x−0.84 μm,R2=0.89; purple:y=0.53x−0.99 μm,R2=0.85; black:y=0.03x+0.94 μm,R2=0.09; grey:y=0.31x+1.25 μm,R2=0.57. (b) The cluster size ofbcdDNA FISH dots against nurse cell nuclear diameter in two inbred lines. SeeSupplementary Fig. 6for spatial properties of gene loci in follicle cells. Figure 3: Expansion of gene locus clusters in expanding nurse cell nuclei. ( a ) Scatter plots of the observed cluster size for individual gene loci ( bcd , nos or Cp , shown in blue, red and purple, respectively), or the observed distance between two clusters ( bcd - nos or bcd - Cp , shown in black and grey, respectively), against nurse cell nuclear diameter (see Methods for definition of cluster size and distance between clusters). Data are from WT egg chambers at stages 6~10 A. Solid lines are linear fits. Blue: y =0.54 x −0.92 μm, R 2 =0.86; red: y =0.54 x −0.84 μm, R 2 =0.89; purple: y =0.53 x −0.99 μm, R 2 =0.85; black: y =0.03 x +0.94 μm, R 2 =0.09; grey: y =0.31 x +1.25 μm, R 2 =0.57. ( b ) The cluster size of bcd DNA FISH dots against nurse cell nuclear diameter in two inbred lines. See Supplementary Fig. 6 for spatial properties of gene loci in follicle cells. Full size image To investigate the spatial relationship between clusters of different gene loci on a chromosome, we analysed double-FISH data for bcd paired with either nanos ( nos ) or a chorion protein gene locus ( Cp , see Methods) in WT embryos. The detected clusters for nos or Cp loci expand similarly to those of bcd inside nurse cell nuclei, supportive of volumetric expansion ( Fig. 3a ). However, between-cluster expansion ( bcd - nos or bcd - Cp ) exhibits properties suggesting that they are subject to constraints sensitive to the intervening DNA length ( Fig. 3a , black squares and grey diamonds; see Methods for additional details and see Supplementary Fig. 6 for spatial properties of gene loci in follicle cell nuclei). Scaling powers for nuclear DNA and bcd gene copy number Since the bcd gene locus is a part of the entire genome undergoing endoreplication, we first quantified the bulk nuclear DNA in relation to the expansion of the nurse cell nuclear diameter l . We estimated the scaling power for the bulk nuclear DNA n 0 using the fitted slope in a log-log plot ( Fig. 4a ). We obtained n 0 =2.42, 2.27 and 2.50 for WT, large- and small-egg lines, respectively (95% confidence intervals are: 2.32~2.51, 2.04~2.50 and 2.22~2.77). Using all data pooled, n 0 =2.43 (95% confidence interval (CI)=2.20~2.66). 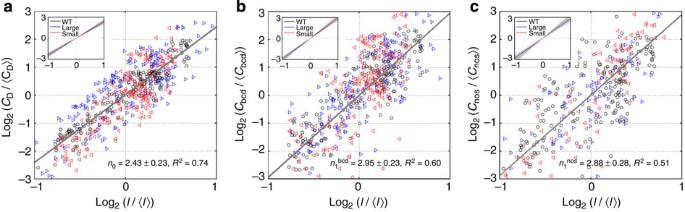Figure 4: Scaling power estimations for bulk nuclear DNA and gene copy numbers in nurse cells. (a–c) Log-log plots for genome polyploidy equivalent (a),bcdgene copy number (b) ornosgene copy number (c), against nurse cell nuclear diameter. Solid line is linear fit, with scaling power, 95% CI andR2shown. Inset shows fitting of data from individual lines. For WT (shown in black),n0=2.42±0.09,R2=0.91;n1bcd=2.82±0.20,R2=0.80;n1nos=2.83±0.22,R2=0.76. For the large-egg line (shown in blue):n0=2.27±0.23,R2=0.67;n1bcd=3.10±0.31,R2=0.67;n1nos=2.79±0.44,R2=0.45. For the small-egg line (shown in red):n0=2.50±0.27,R2=0.74;n1bcd=2.93±0.45,R2=0.60;n1nos=3.14±0.43,R2=0.78. Figure 4: Scaling power estimations for bulk nuclear DNA and gene copy numbers in nurse cells. ( a – c ) Log-log plots for genome polyploidy equivalent ( a ), bcd gene copy number ( b ) or nos gene copy number ( c ), against nurse cell nuclear diameter. Solid line is linear fit, with scaling power, 95% CI and R 2 shown. Inset shows fitting of data from individual lines. For WT (shown in black), n 0 =2.42±0.09, R 2 =0.91; n 1 bcd =2.82±0.20, R 2 =0.80; n 1 nos =2.83±0.22, R 2 =0.76. For the large-egg line (shown in blue): n 0 =2.27±0.23, R 2 =0.67; n 1 bcd =3.10±0.31, R 2 =0.67; n 1 nos =2.79±0.44, R 2 =0.45. For the small-egg line (shown in red): n 0 =2.50±0.27, R 2 =0.74; n 1 bcd =2.93±0.45, R 2 =0.60; n 1 nos =3.14±0.43, R 2 =0.78. Full size image To estimate n A using an independent method that is specific to the bcd gene locus, we determined the relationship between bcd gene copy number and nurse cell nuclear diameter l . We obtained the scaling power of the bcd gene copy number n 1 =2.82, 3.10 and 2.93, 2.95 for WT, large-egg line, small-egg line and three lines pooled, respectively ( Fig. 4b ; 95% CI=2.62~3.03, 2.78~3.41 2.48~3.39 and 2.72~3.18). These results document that n 1 is a maternal property that is insensitive to size of the future egg ( n 1 of the large-egg line is within 95% CI of that of the small-egg line and vice versa ). They support the deduced relationship in equation (3) where n A is defined fundamentally by rate constants of the maternal processes of bcd gene copy number expansion and tissue expansion. To determine whether n 1 obtained for the bcd gene locus is reflective of a general property of an expanding egg chamber in the ovary as postulated ( Supplementary Note 2 ), we measured the scaling power for the locus of nos , another nurse cell-expressing gene. We obtained n 1 =2.83, 2.79, 3.14 and 2.88 in WT, large-egg line, small-egg line and three lines pooled, respectively ( Fig. 4c , 95% CI=2.61~3.06, 2.35~3.23, 2.71~3.57 and 2.65~3.11), values consistent with those measured on bcd . bcd gene copy number at the peak time during oogenesis At stage 10 of oogenesis, nurse cell nuclei reach their peak size [40] . We estimate that a WT stage-10A egg chamber contains a total of 6.3±1.2 × 10 3 copies of the bcd gene in 15 nurse cells combined ( Fig. 2f ; see Fig. 2e legend for estimated genome polyploidy number at the same stage). We note that this peak bcd gene copy number is very similar to the total number of nuclei of a cellularizing blastoderm embryo. A large number of bcd gene templates in an egg chamber would ensure a reliable production of bcd mRNA to be deposited to the egg as seen in the embryo [23] , [29] , [48] . For the large- and small-egg inbred lines, this number is 6.8±1.4 × 10 3 and 5.6±1.1 × 10 3 , respectively. These results document a direct divergence in bcd gene template number in nurse cells of the inbred lines despite the fact that they had been selected based solely on the size of the eggs laid [39] . Measurements of n 2 and n 3 in embryos To further evaluate equation (3), we measured n 2 and n 3 , the scaling power for bcd mRNA and Bcd protein, respectively, in embryos from the inbred lines that offered an enhanced size spread for effective analysis ( Fig. 1b ). We obtained n 2 =2.70 ( R 2 =0.86, 95% CI=2.36~3.04) and n 3 =3.03 ( R 2 =0.71, 95% CI=2.00~4.06; see Supplementary Table 2 for idealized and measured parameters of a full morphogen gradient model). Fig. 5a shows an overlay of measurements for all three molecular species within the linear chain. Supportive of equation (3), datapoints from these independent measurements congregate towards a consensus slope ( Fig. 5a ). Since endoreplication is a regulated process during oogenesis [45] , [49] , [50] , a consensus of n A ~3 suggests that DNA replication for nurse cell-expressing genes is coupled with nuclear volume expansion. 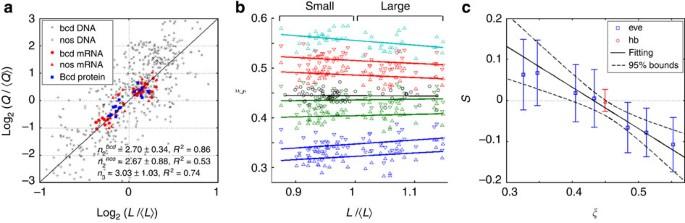Figure 5: Scaling power measurements in embryos and evaluations of model predictions. (a) Superimposed plots showing scaling power measurements in the two inbred lines; also shown is a reference line with a slope of 3. Datapoints forbcdDNA,nosDNA,bcdmRNA,nosmRNA and Bcd protein are shown as x marks, crosses, circles, diamonds and squares, respectively. (b) Scatter plot of relative positions ofhb(black) or the anterior 7eve(coloured) expression boundaries in embryos from these inbred lines (seeSupplementary Fig. 7for a display showing alleveboundaries). Colour code forevedata: blue, green, red and magenta for expression stripes 1–4, respectively, with upright and downward triangles representing anterior and posterior boundaries, respectively. (c) Measured values of scaling coefficientS, estimated as the slope of a regression line (solid lines inb), are plotted as a function of boundary positionξ. Error bars represent 95% CI of each fitted slope. Results forhbandeveare shown in red and blue, respectively. Solid line shown is a linear fit for the selected boundaries (see text;R2=0.94), and dashed lines are 95% prediction bounds of this fit. In another linear fit using boundaries within a wider range of the embryo (hband the first through seventh ofeve), we obtained consistent estimates (ξC=0.422 andnA=2.13) that likely have also incorporated the impact of terminal system inputs on boundaries that are closer to the anterior pole24,51. Extended discussion about scaling coefficientS: Under its current definition (see text),S=0 denotes perfect scaling of a gene’s expression boundary. IfS<0 orS>0, the boundary is either under- or overscaled, respectively. This evaluation is consistent with a previous analysis16performed under the framework of a differently defined scaling coefficientSBerg, as dictated by the relationshipS=ξ(SBerg−1). Figure 5: Scaling power measurements in embryos and evaluations of model predictions. ( a ) Superimposed plots showing scaling power measurements in the two inbred lines; also shown is a reference line with a slope of 3. Datapoints for bcd DNA, nos DNA, bcd mRNA, nos mRNA and Bcd protein are shown as x marks, crosses, circles, diamonds and squares, respectively. ( b ) Scatter plot of relative positions of hb (black) or the anterior 7 eve (coloured) expression boundaries in embryos from these inbred lines (see Supplementary Fig. 7 for a display showing all eve boundaries). Colour code for eve data: blue, green, red and magenta for expression stripes 1–4, respectively, with upright and downward triangles representing anterior and posterior boundaries, respectively. ( c ) Measured values of scaling coefficient S , estimated as the slope of a regression line (solid lines in b ), are plotted as a function of boundary position ξ . Error bars represent 95% CI of each fitted slope. Results for hb and eve are shown in red and blue, respectively. Solid line shown is a linear fit for the selected boundaries (see text; R 2 =0.94), and dashed lines are 95% prediction bounds of this fit. In another linear fit using boundaries within a wider range of the embryo ( hb and the first through seventh of eve ), we obtained consistent estimates ( ξ C =0.422 and n A =2.13) that likely have also incorporated the impact of terminal system inputs on boundaries that are closer to the anterior pole [24] , [51] . Extended discussion about scaling coefficient S : Under its current definition (see text), S =0 denotes perfect scaling of a gene’s expression boundary. If S <0 or S >0, the boundary is either under- or overscaled, respectively. This evaluation is consistent with a previous analysis [16] performed under the framework of a differently defined scaling coefficient S Berg , as dictated by the relationship S = ξ ( S Berg −1). Full size image Experimental evaluation of predictions of the TEM 3 S model We now consider morphogen action in instructing gene expression patterns in system P . If M at a gene’s expression boundary ( ξ ) is fixed, d M =(∂ M /∂ ξ )d ξ +(∂ M /∂ L )d L =0, applying equation (2) and the exponential function of M leads to where d ξ /(d L / L ) quantifies directly how well the fluctuations in L are corrected at ξ . We thus define S =d ξ /(d L / L ) as the scaling coefficient of an expression boundary (see legend to Fig. 5 for additional details). Equation (4) makes three broad predictions about gene expression patterns in embryos if morphogen production (originating from maternal tissue expansion) and action could be recapitulated by the TEM 3 S model: (1) there is a position, ξ C , exhibiting perfect scaling, (2) there is overscaling when ξ < ξ C and (3) there is underscaling when ξ>ξ C . To evaluate these predictions, we performed mRNA FISH experiments to obtain the expression profiles of hunchback ( hb ) and even-skipped ( eve ) in embryos from the two inbred lines (Methods). As shown in Fig. 5b and Supplementary Fig. 7c , the hb boundary ( ξ =0.450) and the fourth boundary of eve ( ξ =0.433) in these embryos are closest to being perfectly scaled: S =−0.005 and 0.005, respectively, whereas the more anteriorly positioned eve boundaries are progressively overscaled. These results support qualitatively the first two predictions. The third prediction is not fully supported since the predicted, progressively worsening underscaling is disrupted at ξ ~0.6 causing a trend reversal ( Supplementary Fig. 7c ), suggesting that patterning decisions in this part of the embryo ( ξ >0.6) are also sensitive to other inputs and regulatory mechanisms [24] , [27] , [51] , [52] . To evaluate our data quantitatively, we linearly fitted S to ξ for boundary positions of hb and the third through sixth of eve ( Fig. 5c legend). This analysis is based on an explicit assumption that these selected boundaries are specified solely by the Bcd gradient input in an idealized system P depicted by TEM 3 S. Using experimentally measured Γ =6.2 (see Supplementary Table 2 for other measurements), we obtained ξ C =0.431 and n A =2.64. In essence, these two values represent the theoretically predicted properties of the embryos should they have followed explicitly the stated model, given the observed expression boundaries. Importantly, n A =2.64 derived that this way is consistent with the values obtained from direct measurements in embryos on the actual molecular species in the linear chain (within 95% CI of n 2 and n 3 ), further supporting TEM 3 S-derived predictions about the patterning outcomes in the specified part of the embryo. Our TEM 3 S model provides a unified view on the properties of maternal morphogen gradients and embryonic patterning from both mechanistic and evolutionary perspectives. Extending our previous findings [14] , [23] , [25] , [29] , [53] , [54] , [55] , [56] , [57] , [58] , [59] , [60] of a faithful input–output relationship between the Bcd input and the expression of its direct target gene hb , our current results ( Fig. 5b black) show that this regulatory relationship can be recapitulated largely by the TEM 3 S model. This particular relationship is likely reflective of the working of active mechanisms to allow hb to respond primarily to the Bcd gradient input [58] , [59] . Thus, the performance objective of attaining a critical position by a maternal morphogen gradient may also be displayed directly by the expression boundaries of, at least in some cases, its target genes. In an idealized TEM 3 S model, a patterning system benefits from having a critical position at the midpoint to allow it to receive the highest overall scaling information derived from the maternal morphogen gradient ( Supplementary Note 1 ). There are evolutionary implications for the existence of a critical position that coincides with the expression boundary of a direct Bcd target gene(s) known to have essential functions [61] , [62] , [63] . Equation (2) indicates that a meaningful critical position is achievable only if the system attribute Γ and the scaling power of the amplitude n A are properly balanced with one another. Given that n A has a finite value dictated fundamentally by the dynamic properties of system E and thus is insensitive to egg size per se (see Fig. 5a and Supplementary Fig. 2 ), evolution of dipteran species with drastically divergent egg sizes would have to be operated under the selection pressure to preserve Γ ( Supplementary Note 1 ). In other words, under the TEM 3 S framework, maintaining scaled and robust embryonic patterning within a species also commanded—barring a regulatory network rewiring—co-evolution of egg size and Bcd gradient properties across different species to preserve the system attribute Γ . This prediction is supported by available data [30] . From the perspective of developmental biology, our TEM 3 S model provides a quantitative framework to evaluate the relationship between tissue growth and tissue specification under temporal logic c . Importantly, it unifies events taking place in two distinct stages of an animal’s life cycle, maternal tissue expansion and embryonic patterning. Under this framework, a robust and scaled patterning outcome of the embryo has a dynamic underpinning that is also inherent to the life cycle itself. Our results show that, meanwhile, the fundamental processes governing maternal tissue expansion impose quantifiable limits to how a developmental programme under temporal logic c can be constructed ( Supplementary Fig. 2 and Supplementary Note 1 ). The other two types of temporal logics ( Fig. 1a ) must likely come with their own limits in connecting their respective expansion and patterning systems [13] , [20] , [64] , [65] , [66] , [67] . These limits together help to shape the forms of life on both ontogenetic and phylogenetic timescales. Our current study also contributes to a broader on-going debate about the fundamental rules in biological scaling. Our results show that, consistent with the fact that parts of the genome are under-replicated in nurse cells [44] , [49] , the scaling power of the bulk nuclear DNA contents n 0 is smaller than that of bcd gene copies n 1 ( Fig. 4a ) and approaches 2.25, the predicted value of the ¾-power scaling rule [1] , [2] . It remains to be known which of the scaling powers, n 0 or n 1 , is the primary indicator for the fundamental mechanisms regulating endoreplication in nurse cells. A precise answer to this question will advance our knowledge of biological scaling at the level of cell cycle control in relation to nuclear size (see Supplementary Fig. 8 , Supplementary Table 3 and Supplementary Note 3 for effects of expansion anisotropy on n A estimations). However, this layer of inquiry will not affect our current conclusion that the core quantity of the TEM 3 S model, n A , has a finite value that can be approximated—through independent measurements—by an effective isometric scaling power relationship. Our quantification of the bcd gene copy number in nurse cells reveals a peak value that resembles the peak number of nuclei in the blastoderm embryo. It is currently unknown whether this resemblance is purely coincidental. When considered in isolation, each value quantities the peak of an exponential expansion process. However, when considered together, they are system-level quantities that are integral to the biology of a mother and her future embryos. It remains to be investigated whether and if so, how, these particular quantities—and their relationship—might have been influenced by evolution. Drosophila melanogaster strains All flies used in this study were raised on standard cornmeal-based media at 25 °C and 60% humidity. w 1118 flies were used as the WT. Two inbred lines, no. 2.46.4 and no. 9.17.1, which have large or small eggs and are referred to as the large-egg line and small-egg line, respectively, were as described [23] . These lines had been derived from an artificial selection and inbreeding process on the basis of the selected traits of egg size extremes [39] and were kindly provided by Cecelia Miles and Martin Kreitman. For each given set of experiments involving these two lines, all experimental and imaging procedures were performed on a side-by-side basis to permit direct comparisons. DNA FISH in Drosophila ovaries Our whole-mount DNA FISH procedure for the ovary was adapted from laboratory protocols of Allan Spradling [46] and Terry Orr-Weaver [68] . Briefly, newly eclosed female flies were cultured on wet yeast for 2 days and transferred to fresh wet yeast for another day. On the fourth day, ovaries were dissected in 400-μl 1 × PBS (137 mM NaCl, 2.7 mM KCl, 10 mM Na 2 HPO 4 and 2 mM KH 2 PO 4 ), fixed in 4% paraformaldehyde with 0.5% Triton X-100 for 15 min, washed with 2 × SSCT (300 mM NaCl, 30 mM Sodium Citrate and 0.1% Tween-20) three times and treated with 10 μg ml −1 RNaseA and RNaseT in 2 × SSCT at room temperature for 30 min. For prehybridization, the ovaries were transferred step-wise to 2 × SSCT with increasing concentrations of formamide (0, 20, 40 and 50%) and incubated in fresh 2 × SSCT with 50% formamide at 37 °C for 1 h. The ovaries were then mixed with 40 μl of probe solution consisting of 36 μl 1.1 × Hybridization Buffer (10% Dextran Sulfate, 3 × SSC and 50% Formamide) and 4 μl probe (400 ng), denatured at 96 °C for 8 min and chilled on ice for 5 min, before overnight (~16 h) incubation at 37 °C. After hybridization, ovaries were washed with 2 × SSCT with 50% formamide at 37 °C for 4 × 15 min, and transferred step-wise to 2 × SSCT with 50, 40, 20 and 0% formamide, and finally washed with 2 × SSCT for 3 × 10 min. During the last washing step, the ovaries were brought to room temperature and further incubated with 4′,6-Diamidino-2-phenylindole dihydrochloride (DAPI, 1:1,000 dilution, Sigma) and Alexa Fluor 555-conjugated WGA (WGA-555 1:300 dilution, Invitrogen) at room temperature for 10 min. After washing with 2 × SSCT for 5 × 10 min, egg chambers were mounted in Vectashield reagent (Vector Laboratories) before imaging. Coverslip was gently pressed during mounting, when appropriate, to reduce excessive tissue thickness. Probe preparations for DNA FISH Probes for DNA FISH were prepared by nick translation using either the FISH Tag DNA Green Kit (Alexa Fluor 488, Life Technology) or the FISH Tag DNA Red Kit (Alexa Fluor 594, Life Technology) according to the manufacturer’s instructions. Primer sequences to generate the DNA templates are listed in Supplementary Table 1 . Each probe set contains six to seven individual probes (~1.3 to ~1.7 kb each) designed to span >16 kb surrounding the target gene body but excluding the coding sequences. Unlike bcd and nos , which are unique genes, there are four clusters of the chorion gene within the genome [68] , DAFC-7F on chromosome X, DAFC-30B on chromosome X, DAFC-62D on chromosome 3 L and DAFC-66D on chromosome 3 L. Our Cp probe set was designed to detect the 66D locus on 3 L including Cp18 , Cp15 , Cp19 and Cp16 . All PCR products (from genomic DNA) used for generating probes were verified using gel electrophoresis to be of expected size as designed. Confocal imaging and documentation of intensity linearity Images were acquired on a Nikon A1Rsi Confocal microscope equipped with a × 20 objective with × 3 digital zoom. All confocal images were captured under identical settings, with the pinhole size at 1.2 AU and the amplifier offset at 0. A series of gain values (photomultiplier voltage (PMV)) were tested to determine the linear range of the pixel intensity for each channel ( Supplementary Fig. 5 ). These linearity tests were on the basis of entire images to ensure that the linearity documented in Supplementary Fig. 5 is applicable to the entire intensity range including the signals from nurse cells. Images captured were 8-bit in depth and 1,024 × 1,024 in the xy resolution. The z -step size was set to match the xy pixel size (0.21 μm). For egg chambers that cannot be captured by a single image because their size exceeded the imaging field, 2 × 2 images with 15% overlap were captured and stitched. Defining the oogenesis stage of each egg chamber We followed established criteria to assign an egg chamber to one of the 14 stages of oogenesis [40] . We focused on stages 3~10 A for optimal size range and measurement reliability. We used the following morphological landmarks to assign an egg chamber to a developmental stage. At stage 3, the loss of oocyte nucleolus can be easily detected in the DAPI channel. At stage 4, the egg chambers are oval-shaped and DAPI staining shows a well-resolved bulbous structure in the nurse cell nuclei. The bulbous structure becomes dissolved at stage 5 and, concurrently, the homologous chromosomes begin to disassociate with multiple FISH dots becoming detectable in a nurse cell nucleus; dispersion of FISH dots continues into stage 6 as reported [46] . At stage 7, the egg chamber becomes elongated, which accompanies the onset of polyploidation and enlargement of follicle cells. Egg yolk becomes first detectable at stage 8; this stage also marks the start of follicle cell migration, a process that continues into stage 9. During stage 9, border cell migration is initiated and the size of the oocyte (measured in length) is ~1/3 to ~1/2 of egg chamber length. The start of stage 10A is marked by the completion of border cell migration to the boundary of oocyte and the oocyte size reaching 1/2 of egg chamber length. Stage 10A ends when centripetal follicle cells begin to migrate. Measuring the egg chamber size For each z -step image, we first generated a mask image combining signals from all channels above a threshold based on Otsu’s method [69] . The length L was defined as the longest distance between two pixels of each egg chamber (that is, the major axis or pseudo AP axis) on the maximum projection of all z -sections. The height H was then defined as the longest distance perpendicular to L on the same projection. L and H were measured automatically using MATLAB (Math Works); for egg chambers that are in physical contact with each other, manual adjustments were made. We performed five repeated measurements to obtain an average and found that a typical measurement error was ~1%. Estimating the detection efficiency of DNA FISH Follicle cells were used to estimate the detection efficiency because of their large numbers and relatively uniform DNA FISH intensities. Among the 2,695 identifiable follicle cell nuclei from 30 w 1118 egg chambers at stages 7~10 A, 2,373 of them had a single bcd fluorescent dot detected, 297 of them had two dots and 25 of them had none. This suggests a detection efficiency of ~99% under our experimental procedure, with a high frequency (~89%) of association between homologous chromosomes in follicle cell nuclei. Similar results were obtained for two other loci analysed in this study, nos and Cp . Before chromosome dispersion, each nurse cell nucleus had on average 0.91±0.27, 0.94±0.33 and 0.89±0.21 identifiable FISH dots for the loci of bcd , nos and Cp , respectively, on the basis of 82 nurse cells analysed (from 10 w 1118 egg chambers at stages 2~5). After dispersion, up to 32 FISH dots were detectable per nurse cell nucleus, with an average of 21.0±6.3, 21.3±6.9 and 21.1±8.0 for bcd , nos and Cp , respectively, on the basis of 335 nurse cells from 39 egg chambers analysed. This suggests an incomplete dissociation of polytene chromosomes in our whole-mount tissues that were processed under conditions to maximally preserve their native spatial features (see also Main text). Measuring the statistics of DAPI and FISH signals Thresholds were determined, on the basis of the following two considerations, to identify nuclei and FISH dots: (1) the intensity threshold was sufficiently high to eliminate false objects arisen from stochastic noise; (2) the threshold was high enough to avoid fusion of neighbouring objects. These two tests led to a stable profile of the number of identified objects against the chosen threshold within a range. Thresholds were then chosen automatically within the stable region where the first-order slope is equal to 0. The sizes and the intensities of nuclei and FISH dots were quantified by two methods. In the first method, the volume of a nucleus or a FISH dot was defined as the number of voxels within each identified object, and the intensity was defined as the aggregated intensity of all voxels within each identified object. Background values of either DAPI or FISH signals were acquired from the mean voxel intensities in regions away from nuclei. In the other method, the centre voxel of each identified object was enclosed by a smallest sphere with a volume ( V ), and the total raw intensity ( I ) was aggregated from all voxels within the sphere. We then fitted data to a two-parameter linear model, I = aC + bV , where C is the polyploidy number (for DAPI) or gene copy number (for FISH); see below for details about data calibration. The choice of shape and size of the enclosing sphere did not alter our conclusions and the linearity between the sizes or the intensities measured by two independent methods further confirmed the reliability of our quantification methods. Measuring the spatial distributions within nuclei The distance between a FISH dot and the nuclear envelope of a follicle cell was measured as the shortest Euclidean distance from any voxel within the FISH dot to any voxel on the boundary of the identified nucleus ( Supplementary Fig. 6 ). The distance between two FISH dots within a follicle cell nucleus was measured as the Euclidean distance between the centre voxels of the two FISH dots ( Supplementary Fig. 6 ). The one-dimensional (1D) size of a cluster of FISH dots of a gene locus was measured as the longest distance between any two dots within the cluster ( Fig. 3a,b ). The distance between the clusters of two gene loci was measured as the Euclidean distance between the weighted centre positions of the two clusters. Two pairs of gene loci (all on chromosome 3) were evaluated for their spatial relationships, and their intervening DNA lengths are: bcd - nos ( Fig. 3a , black squares), 12.4 Mbps (both on 3R); bcd-Cp ( Fig. 3a , grey diamonds) and 19.3 Mbps (on two different arms of chromosome 3). Calibrating the copy numbers of DNA contents and gene locus We used data from the identified follicle cells in stages 7~10-A egg chambers for calibration purposes. The distribution of DAPI intensity of these follicle cells was plot on a log2 scale, which uncovers four well-separated subpopulations. We assigned, as before [45] , the expected 2C, 4C, 8C and 16C, respectively, to each of the four largest subpopulations in the distribution of raw DAPI intensity of follicle cells ( Fig. 2a ). The approximately twofold-DAPI intensity difference between any given two adjacent subpopulations validates this assignment [45] . The boundary intensities between two adjacent subpopulations were specified by the values in the valleys and acquired as the intensity index where the first-order differentiation of the probability density function is 0. In our calibration, we grouped the follicle cells according to their DAPI intensities ( I D ) and their assigned DNA contents expressed as a polyploidy number ( C D ). Then we fitted the data to a two-parameter linear model, I D = a 1 C D + b 1 V D . For DNA FISH data, we assumed that in follicle cells, the copy number of the gene locus ( C g ) is the same as C D and performed the fitting with I g = a 2 C g + b 2 V g . With the parameters a and b obtained for each set of experiments, we converted the detected intensity data to estimates of both the bulk DNA contents expressed as the polyploidy equivalent and the copy number of a gene locus in a nurse cell. See Supplementary Fig. 5 and the confocal imaging section above for discussions about intensity range and linearity documented experimentally. RNA FISH in Drosophila embryos RNA FISH in embryos was performed using fluorescence-labelled probes or digoxigenin-labelled probes detected by an antidig antibody and a fluorescence-labelled secondary antibody [58] . In our current study, probes were prepared from cDNA plasmids or genomic PCR products; for direct fluorescence labelling, the FISH Tag RNA kit (Alexa Fluor 488, Life Technology) was used. Embryos used in bcd and nos mRNA FISH were from 0- to 1-h collections and those used in hb and eve mRNA FISH from 0- to 3- and 0- to 4-h collections, respectively. Imaging was performed under the Zeiss Imager Z1 ApoTome microscope with a Zeiss Plan × 10 Aprochromat objective. Imaging acquisition was performed under linear settings and data analysis (MATLAB, Math Works) was on the basis of fluorescent intensities extracted from the cytoplasmic layer of midsagittal images as a function of AP position (for hb and eve ) [58] or as epifluorescence intensities (for bcd and nos ) [23] . TEM 3 S model and other theoretical considerations Supplementary Notes 1–4 provide a formal presentation of the TEM 3 S model and other related aspects of theoretical considerations. How to cite this article: He, F. et al . Fundamental origins and limits for scaling a maternal morphogen gradient. Nat. Commun . 6:6679 doi: 10.1038/ncomms7679 (2015).